Cracking-assisted photolithography for mixed-scale patterning and nanofluidic applications Cracks are observed in many environments, including walls, dried wood and even the Earth’s crust, and are often thought of as an unavoidable, unwanted phenomenon. Recent research advances have demonstrated the the ability to use cracks to produce various micro and nanoscale patterns. However, patterns are usually limited by the chosen substrate material and the applied tensile stresses. Here we describe an innovative cracking-assisted nanofabrication technique that relies only on a standard photolithography process. This novel technique produces well-controlled nanopatterns in any desired shape and in a variety of geometric dimensions, over large areas and with a high throughput. In addition, we show that mixed-scale patterns fabricated using the ‘crack-photolithography’ technique can be used as master moulds for replicating numerous nanofluidic devices via soft lithography, which to the best of our knowledge is a technique that has not been reported in previous studies on materials’ mechanical failure, including cracking. Standard photolithography techniques produce various micropatterns but are limited to a feature size of approximately a micron [1] . To overcome this limitation, conventional nanolithography techniques such as electron-beam lithography and focused ion-beam are commonly employed [2] . Often, the standard photolithography and nanolithography techniques are used together to create mixed-scale patterns. However, the nanolithography and/or the combination of the two multi-scale lithography techniques show weaknesses in throughput and cost caused by the direct-writing-based nanofabrication processes and scale-up or scale-down lithography processes in series [2] , [3] . Cracks are considered material failures and have never been welcome in micro/nanofabrication processes, but active manipulation of cracking phenomena made it possible to produce various micro and nanoscale patterns, showing remarkable potential for a novel unconventional patterning technique [4] , [5] , [6] , [7] , [8] , [9] , [10] , [11] , [12] , [13] , [14] . However, the cracking-based micro and nanopatterns show several weaknesses and limitations: only one-dimensional (1D) or limited 2D patterns because of the direction of applied stresses [4] , [5] , [6] , [7] , [8] , [9] and the crystallinity of a substrate [11] , respectively; the insufficient controllability of the geometric dimension (for example, width, depth and length) of cracks/patterns caused by the incapability of manipulating the stress strength [6] , [7] , [8] , [10] , [11] , [12] , [13] , [14] ; low success rates in patterning because of unwanted crack formation [4] , [9] , [11] ; low throughput in fabrication because of sequential and multiple fabrication processes [11] , [14] ; incompatibility with other microfabrication processes [5] , [6] , [7] , [10] and low reproducibility by micromoulding and/or soft lithography [10] , [11] , [12] . The most relevant alternatives for cracking-based patterning appear to partially or individually address the weaknesses and limitations [4] , [8] , [9] , [11] . Therefore, a novel technique that can comprehensively and fully address all the weaknesses and overcome the crucial limitations is strongly required for the practical application of crack-based patterns. Here we describe a cracking-assisted photolithography technique that utilizes a non-crystalized, monolithic and organic material (for example, SU-8 photoresist) for the first time and relies only on a standard photolithography process. This innovative technique can produce any desired nanopatterns on the surface of a micropatterned photoresist over large areas, with a high throughput, and with no need for any specific nanofabrication techniques and equipment. Furthermore, the technique allows accurate control of the geometric dimensions of the nanopatterns, thereby resolving the limitations that previous cracking-based techniques were confronted by. As an example of practical application, we demonstrate a nanofluidic device with 1,000 pairs of microchambers that are individually interconnected by a crack-assisted nanochannel; it appears to be impossible to produce the same nanofluidic device by using either the conventional or the unconventional fabrication techniques because of throughput and controllability limits, respectively. However, the technique proposed in this work can produce such a complex nanofluidic device in a single batch process with high reproducibility by soft lithography and with positioning of both the microchannels and nanochannels on the same surface, which is essential for a broad range of nanofluidic applications. Therefore, the ‘crack-photolithography’ technique will provide an unprecedented nanofabrication technique for various nanopatterns and numerous nanofluidic applications. 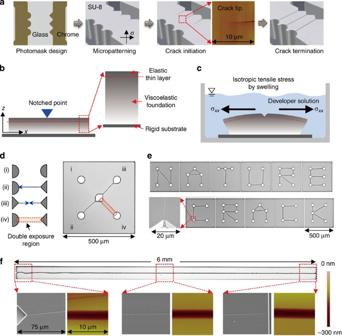Figure 1: Cracking-assisted photolithography. (a) Schematic diagram describing the process, from designing a photomask to fabricating nanopatterns on the surface of micropatterned photoresist. Cracking is initiated and terminated at the previously designed micro-notch structures. The inset is an atomic force microscopy (AFM) image showing a propagating crack tip. (b) The ultraviolet-exposed photoresist consists of an elastic thin layer on a viscoelastic layer on a silicon substrate and exhibits a gradient in cross-linking density along the direction normal to the substrate. (c) The viscoelastic layer swells during the development process, causing the occurrence of tensile stresses in the elastic layer. This two-layered thin film in the presence of tensile stresses generates cracking at the notch, where stresses are more concentrated. (d) The images reveal that not only the shapes of the micropatterns but also the exposure energy can be used to precisely control the initiation and termination of cracking. (e) Controlling the cracking mechanism permits the creation of various nanopatterns, including the words ‘NATURE’ and ‘CRACK’, produced by connecting the nodes with cracking-assisted nanopatterns. (f) Scanning electron microscopy and AFM images of 6-mm long, 2-μm wide and 170-nm deep straight nanopattern. The uniformity of the width and depth throughout the nanopattern is revealed. Mechanism for creating cracking-assisted nanopatterns Figure 1a shows a schematic diagram of the proposed nanofabrication process. Micropatterns with feature sizes of about 5 μm are typically fabricated by using standard photolithography [1] , and using specific stress-concentrating and/or stress-releasing structures in conjunction one can control the initiation, propagation and termination of cracking to create the desired nanopatterns ( Supplementary Fig. 1 ). For example, a sharp notch tends to concentrate stresses more effectively than a blunt one, and causes formation of cracks. In general, cracks are initiated when a stiff and thin elastic layer placed on a viscoelastic underlying layer is subjected to tensile stresses higher than its fracture strength [15] , [16] . In the present work, the elastic and viscoelastic layers were formed by exposing the same spin-coated photoresist (10-μm thick) to ultraviolet light without using the i-line filters recommended by the manufacturer to enable uniform cross-linking throughout the thickness [17] . This delicate process produced a relatively stiff and elastic layer onto a viscoelastic layer with a cross-linking gradient along the direction normal to the substrate, namely a silicon wafer ( Fig. 1b ). Tensile stresses occur naturally in the elastic layer during the development process, causing the viscoelastic layer to swell ( Fig. 1c ) [18] . When the coarsely cross-linked viscoelastic layer absorbs the solvent molecules, it swells isotropically, and consequently, the thin elastic layer above is subjected to an isotropic tensile stress. Once cracking is initiated, it keeps propagating until it reaches a termination structure, whereupon the concentrated stresses are finally released. Thus, a nanoscale crack is successfully created between the initiating notch and the termination structure, as planned during the design stage. Additional details are provided in Supplementary Note 1 . Figure 1: Cracking-assisted photolithography. ( a ) Schematic diagram describing the process, from designing a photomask to fabricating nanopatterns on the surface of micropatterned photoresist. Cracking is initiated and terminated at the previously designed micro-notch structures. The inset is an atomic force microscopy (AFM) image showing a propagating crack tip. ( b ) The ultraviolet-exposed photoresist consists of an elastic thin layer on a viscoelastic layer on a silicon substrate and exhibits a gradient in cross-linking density along the direction normal to the substrate. ( c ) The viscoelastic layer swells during the development process, causing the occurrence of tensile stresses in the elastic layer. This two-layered thin film in the presence of tensile stresses generates cracking at the notch, where stresses are more concentrated. ( d ) The images reveal that not only the shapes of the micropatterns but also the exposure energy can be used to precisely control the initiation and termination of cracking. ( e ) Controlling the cracking mechanism permits the creation of various nanopatterns, including the words ‘NATURE’ and ‘CRACK’, produced by connecting the nodes with cracking-assisted nanopatterns. ( f ) Scanning electron microscopy and AFM images of 6-mm long, 2-μm wide and 170-nm deep straight nanopattern. The uniformity of the width and depth throughout the nanopattern is revealed. Full size image Cracking can be easily controlled either by the shape of the micropattern (decided during mask design), which determines the concentrated stress near notches, or crack tips ( σ c ) or the amount of exposure energy (during fabrication), which influences material properties, including fracture strength ( σ f ). For example, in cases (i) and (iv) of Fig. 1d , cracking was not initiated because stresses were insufficiently concentrated, since the used structure had a rounded shape ( σ c < σ f ), and in addition, the high exposure energy caused a strong cross-linking in the photoresist, further increasing the fracture strength ( σ c < σ f ). Conversely, in cases (ii) and (iii), cracks initiated and propagated in straight lines until terminated by a structure with a rounded shape or until in contact with other cracks ( Supplementary Fig. 2 for crack merging). In addition, we demonstrated that the cracking-assisted nanofabrication technique is capable of creating various nanopatterns with arbitrary trajectories, including words like ‘NATURE’ and ‘CRACK’ ( Fig. 1e ) or long, straight nanochannels (6 mm) with a uniform width (2 μm) and depth (170 nm) ( Fig. 1f ). Control of cracking for mixed-scale patterns We investigated the control of initiation, propagation and termination of cracking by testing various stress-concentrating and stress-releasing microstructures. The experimental results are categorized into three cases: multiple cracks originating from acute notches ( θ N <90°, σ c >> σ f ), single cracks originating from obtuse notches (90°< θ N <148°, σ c > σ f ) and no crack formation around circular notches ( θ N >148°, σ c < σ f ; Fig. 2a and Supplementary Fig. 3 ). It is evident that the acute angles of the isosceles-triangle-shaped notch concentrate stresses more effectively than the obtuse ones. When concentrated stresses are higher than the fracture strength of the photoresist, cracking initiates and propagates until the concentrated stresses at the crack tip are comparable to or lower than the fracture strength. 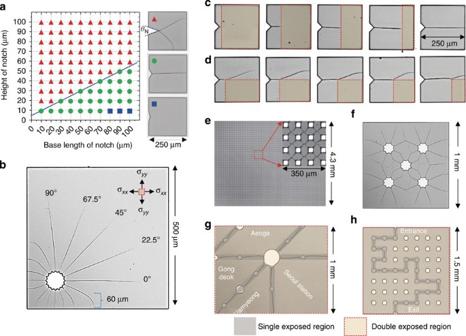Figure 2: Control of cracking for nanopatterns with arbitrary trajectories. (a) Effect of the notch shape on the initiation of cracking. Acute angles tend to initiate more than two cracks, while obtuse angles result in one crack. The blue dashed line indicates the critical angle (90°). The microscopic images on the right show representative types of crack initiation (Supplementary Fig. 3). (b) Isotropic propagation and redirection behaviour of crack tips. (c,d) Prevention and termination of cracking by adjusting the exposure energy. The red dashed boxes indicate the double exposed areas in which no cracking is observed. (e,f) The single exposure process allows production of complex, well-organized and short nanopatterns (lP<1 mm). (g,h) The double exposure process allows production of precisely determined, long nanopatterns such as the Seoul subway map in which micropatterned stations are connected with cracking-assisted nanopatterns (lP>1 mm). More than 400 stations and about 330-km long railway were miniaturized in an area of 4 cm2(Supplementary Figs 6 and 7). Figure 2b shows that cracking can be initiated everywhere and its propagation trajectories may be oriented in any direction because of the amorphous nature of the photoresist and the isotropic tensile stresses. Interestingly, crack tips are redirected and affected by the notch spacing and boundary conditions that are also important factors determining cracking behaviour ( Supplementary Figs 4 and 5 ). Figure 2: Control of cracking for nanopatterns with arbitrary trajectories. ( a ) Effect of the notch shape on the initiation of cracking. Acute angles tend to initiate more than two cracks, while obtuse angles result in one crack. The blue dashed line indicates the critical angle (90°). The microscopic images on the right show representative types of crack initiation ( Supplementary Fig. 3 ). ( b ) Isotropic propagation and redirection behaviour of crack tips. ( c , d ) Prevention and termination of cracking by adjusting the exposure energy. The red dashed boxes indicate the double exposed areas in which no cracking is observed. ( e , f ) The single exposure process allows production of complex, well-organized and short nanopatterns ( l P <1 mm). ( g , h ) The double exposure process allows production of precisely determined, long nanopatterns such as the Seoul subway map in which micropatterned stations are connected with cracking-assisted nanopatterns ( l P >1 mm). More than 400 stations and about 330-km long railway were miniaturized in an area of 4 cm 2 ( Supplementary Figs 6 and 7 ). Full size image Figure 2c shows that the exposure energy affects cracking because the local fracture strength of the double exposed region (~250 mJ cm −2 ) is higher than that of the single one (~125 mJ cm −2 ). Overall, there are three ways to stop the propagation of cracking: first crack-terminating structures (local relaxation of σ c ); second spatially increased exposure energy (local enhancement of σ f ); and last removing the photoresist from the developer (throughout stress removal). The first two methods are useful to selectively terminate cracking, while the last one is used for the immediate termination of all propagating cracks. Also, a propagating crack tip can be redirected by forming spatially non-uniform fracture strength which can be achieved by using different amounts of exposure energy, resulting in a crack tip that cannot propagate straight, instead of detouring to the open boundary ( Fig. 2d ). It is worth noticing that single exposure is appropriate to generate complex but well-organised, short nanopatterns throughout micropatterns (propagation length, l P <1 mm) ( Fig. 2e,f ), while double exposure allows selective and precise formation of long nanopatterns along the desired paths ( l P >1 mm; Fig. 2g,h ). This is because the single exposed photoresist is more vulnerable to molecular level defects that can act as notches to initiate unwanted cracking, whereas the double exposed photoresist enables the formation of cracking onto the single exposed region only, preventing the occurrence of unwanted cracking. All these characteristics allow the production of nanopatterns that could not be achieved using either conventional techniques showing low throughput and requiring high cost or unconventional techniques depending on a crystallized substance [11] and/or applied anisotropic tensile stresses [4] , [5] , [8] , [9] ( Supplementary Figs 6 and 7 ). Control of propagation velocity and crack dimension The cracking behaviour was characterized from the viewpoint of propagating distances/velocities and geometric dimensions of cracks under various photolithography conditions. First of all, the propagating distances are proportional to the development time and decrease with increasing exposure energy ( Fig. 3a and Supplementary Fig. 8 ). This is because an increased exposure energy causes an increase in the material failure strength, thanks to stronger cross-linking [19] . We note that the maximum crack length may not be limited but the ultraviolet exposure time needs to increase to reduce the crack width and depth, resulting in the increase of development time. Therefore, the development time can be a limiting factor for long cracks. Surprisingly, the propagating velocities were substantially slower (1–22 μm min −1 ) than those reported in previous studies [4] , [11] , [20] , enabling us to precisely control the length of cracks ( Supplementary Fig. 9 and Supplementary Note 2 ). In addition, the width of the fully formed cracks varied between 0.5 and 2.7 μm, their depth between 40 and 190 nm. Both dimensions are inversely proportional to the exposure energy ( Fig. 3b,c and Supplementary Fig. 10 ) because the volume expansion due to swelling decreases as the cross-linking density increases [18] . We also found that the cracks tend to reach a constant width-to-depth ratio of about 10 (for example, 130-nm deep and 1.3-μm wide; Fig. 3d and Supplementary Fig. 11 ). This means that the crack surface in the photoresist is suitable for the fabrication of uniform nanoslit structures commonly found in nanofluidic applications [21] . The surface profiles of the propagating crack tips are presented in Supplementary Fig. 12 . 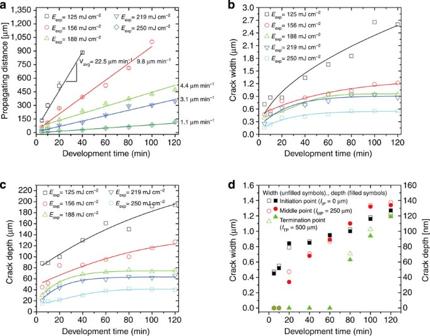Figure 3: Characterization of cracking behaviour and geometry of cracks. (a) The propagation distances and velocities (slopes) were measured using microscopic images of the cracks produced on single exposure photoresist micropatterns. The error bars correspond to the s.d. of 10 different cracks on a single wafer. The measurement of the distances was limited to 1 mm to avoid the unwanted initiation of cracking. The data points are fitted using a linear approximation. (b,c) Width and depth of the cracks. The data points are fitted using asymptotic functions (y=a+b×cx, wherea,bandcare constants). (d) Width (unfilled symbols) to depth (filled symbols) ratio along the crack propagating direction. The width and depth of the cracks propagating for up to 500 μm were measured as a function of the development time in three regions-of-interest, including the initiation point (lIP=0 μm), a middle point (lMP=250 μm) and a termination point (lTP=500 μm), resulting in a ratio of 10. All the data were obtained from AFM images for high accuracy (Supplementary Figs 10 and 11). Figure 3: Characterization of cracking behaviour and geometry of cracks. ( a ) The propagation distances and velocities (slopes) were measured using microscopic images of the cracks produced on single exposure photoresist micropatterns. The error bars correspond to the s.d. of 10 different cracks on a single wafer. The measurement of the distances was limited to 1 mm to avoid the unwanted initiation of cracking. The data points are fitted using a linear approximation. ( b , c ) Width and depth of the cracks. The data points are fitted using asymptotic functions ( y = a + b × c x , where a , b and c are constants). ( d ) Width (unfilled symbols) to depth (filled symbols) ratio along the crack propagating direction. The width and depth of the cracks propagating for up to 500 μm were measured as a function of the development time in three regions-of-interest, including the initiation point ( l IP =0 μm), a middle point ( l MP =250 μm) and a termination point ( l TP =500 μm), resulting in a ratio of 10. All the data were obtained from AFM images for high accuracy ( Supplementary Figs 10 and 11 ). Full size image Furthermore, not unexpectedly, it is very important to investigate the effect of film thicknesses on cracking behaviour and crack dimension. As shown in Fig. 4 , the thinner ( d SU-8 =11.5 μm, Fig. 4a ) film shows slower propagation velocities ( Fig. 4c ) and smaller aspect ratios ( Fig. 4d ) than the thicker one ( d SU-8 =17.3 μm, Fig. 4b ) under the same photolithography conditions. This can be attributed to the fact that the thinner film can be more densely cross-linked than the thicker film under the same exposure energy ( E exp =188 mJ cm −2 ). In addition, the thicker (more coarsely cross-linked) film may cause stronger tensile stresses by absorbing more solvent molecules than the thinner film. In this context, it is noted that a wide range of aspect ratios of cracks can be obtained by manipulating different combinations of the film thickness and the exposure energy, showing high potential for producing various nanopatterns in conjunction with micropatterns simultaneously. 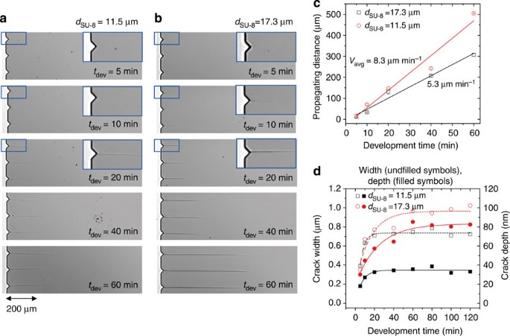Figure 4: Effect of film thickness on cracking behaviour. (a,b) Microscopic images of cracks created on the surface of micropatterned photoresist with film thicknesses (dSU-8) of 11.5 and 17.3 μm, respectively. (c) Quantification of propagation distances and corresponding velocities. The linear guide lines were obtained by using a least-square method. (d) Quantification of the width and depth of the cracks as a function of development time. The data points were fitted using asymptotic functions (y=a+b×cx, wherea,bandcare constants). Figure 4: Effect of film thickness on cracking behaviour. ( a , b ) Microscopic images of cracks created on the surface of micropatterned photoresist with film thicknesses ( d SU-8 ) of 11.5 and 17.3 μm, respectively. ( c ) Quantification of propagation distances and corresponding velocities. The linear guide lines were obtained by using a least-square method. ( d ) Quantification of the width and depth of the cracks as a function of development time. The data points were fitted using asymptotic functions ( y = a + b × c x , where a , b and c are constants). Full size image Fabrication of master moulds for nanofluidics As an application of the proposed technique, we developed a nanofluidic device consisting of 1,000 nanochannels (132-nm deep, 1.4-μm wide and 200-μm long), each one connecting 2 microchambers ( Fig. 5a–f and Supplementary Movie 1 ). The negatively patterned SU-8 mould was replicated using polyurethane acrylate (PUA) for a positive mould, which in turn was replicated using polydimethylsiloxane (PDMS; Supplementary Fig. 13 ). The success rate of the crack-assisted nanochannel fabrication was an astonishing 99.9% ( Supplementary Video ). It is worth noticing that an SU-8 mould can be used for several tens of PUA replications, and each PUA mould can be used for several hundreds of PDMS replications [22] . This shows the unique capability of the proposed technique to form nanopatterns with high throughput over large areas and to provide an extremely reproducible fabrication method for soft lithography [23] ( Supplementary Note 3 ). Using the PDMS replica devices, we demonstrated that the transport of fluorescein isothiocyanate (FITC) is freely diffused from one microchamber to the opposite one, although 1 μm fluorescent particles could not penetrate the nanochannel ( Fig. 5g ). This is very important because accurate control of the transport of small molecules in nanofluidic devices is crucial for various biological and physicochemical assays and applications [24] , [25] . An applied electric potential was also used to test the rapid electrokinetic migration of FITC, and we demonstrated that the nanochannel was very robust and reliable even under oscillating electric potentials ( Fig. 5h,i ). Because of the high hydraulic resistance of the nanochannel, pressure-driven flow was negligible, thus demonstrating that the nanochannel could not only play a key role in nanofluidic devices but also replace nanoporous membranes widely used in micro and nanofluidic devices [25] . Given that a nanochannel array can be easily integrated with other microfluidic components on the same layer, single-layered, membrane-free micro and nanofluidic devices may potentially be developed using cracking-assisted photolithography. 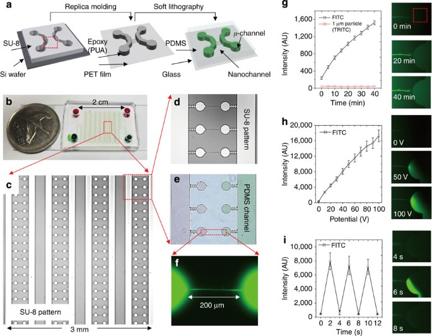Figure 5: Nanofluidic application of cracking-assisted nanopatterns. (a) Fabrication processes: negative micropatterns with cracks are replicated with PUA for a positive mould, which is in turn replicated with PDMS for a single-layered, nanochannel-integrated nanofluidic device. (b) The nanofluidic device has 1,000 pairs of microchambers connected through nanochannels for the transport of small molecules. (c) Microscopic image of an SU-8 mould. (d) Details of micropatterns for chambers and cracks for nanochannels. (e) Microscopic image of a PDMS replica device filled with solutions of green (right) and red (left) dyes. (f) Fluorescent image showing mass transport by diffusion from left to right along a nanochannel. (g–i) Quantitative and qualitative characterization of mass transport: transient diffusion, electrokinetic migration and oscillatory control of the migration of small molecules by electric potentials throughout a nanochannel (Supplementary Fig. 14). The average values and error bars were obtained from triplicate experiments. Figure 5: Nanofluidic application of cracking-assisted nanopatterns. ( a ) Fabrication processes: negative micropatterns with cracks are replicated with PUA for a positive mould, which is in turn replicated with PDMS for a single-layered, nanochannel-integrated nanofluidic device. ( b ) The nanofluidic device has 1,000 pairs of microchambers connected through nanochannels for the transport of small molecules. ( c ) Microscopic image of an SU-8 mould. ( d ) Details of micropatterns for chambers and cracks for nanochannels. ( e ) Microscopic image of a PDMS replica device filled with solutions of green (right) and red (left) dyes. ( f ) Fluorescent image showing mass transport by diffusion from left to right along a nanochannel. ( g – i ) Quantitative and qualitative characterization of mass transport: transient diffusion, electrokinetic migration and oscillatory control of the migration of small molecules by electric potentials throughout a nanochannel ( Supplementary Fig. 14 ). The average values and error bars were obtained from triplicate experiments. Full size image The proposed technique appears to be the simplest and most controllable methodology among the fabrication techniques based on materials failure [21] , and presents many advantages such as cost reduction, time optimization, suitability for large areas and simultaneous production of micropatterns and nanopatterns. In addition, the technique affords: a wide range of nanochannel dimensions with depths varying between 40 and 190 nm, widths between 0.5 and 2.7 μm and lengths between 10 and 10,000 μm; perfect compatibility with conventional photolithography without any need for additional nanolithography processes and equipment; and practical applications such as mixed-scale master moulds for micro and nanofluidic devices. Furthermore, the technique can be distinguished from the most relevant alternatives [4] , [8] , [9] , [11] from the viewpoint of perfect 2D nanopatterning; accurately manipulated isotropic stresses; simultaneous micro/nanopatterning in a monolithic material; complete suppression of unwanted cracking; whole and complete controllability of crack dimension, termination and redirection and a versatile experimental platform for studying the fundamental physics and mechanics of materials failure [16] . Hence, the proposed ‘crack-photolithography’ will not only open new opportunities for advancement of nanopatterning technologies but also revolutionize the development of novel micro and nanofluidic devices. Cracking-assisted photolithography process SU-8 (2010, MicroChem, USA) was spin coated on a silicon wafer at 3,000 r.p.m. for 30 s to obtain a 10-μm thick photoresist film. After soft baking on a hotplate (95 °C) for 3 min, the SU-8 was exposed to ultraviolet light using the first photomask and a mask aligner (MA6, Suss MicroTec, Germany). No optical filters were used to create a cross-linking gradient in the direction normal to the substrate. Then, the SU-8 was post-exposure baked on a hotplate (95 °C) for 3 min before developing. For a single exposure (photomask) process, the SU-8 was maintained in fresh SU-8 developer solution (MicroChem, USA) for more time than required by the specifications, with the process time depending on the crack length and varying between 2.5 and 120 min. For a double exposure (photomask) process, the SU-8 was firstly developed for 2.5 min and then removed from the developer solution and rinsed thoroughly. Then, the SU-8 micropatterns were exposed again to ultraviolet light using the second photomask, baked as above and developed for long as necessary. The first photomask was used to produce micropatterns with notch structures, while the second one was optionally used, not only to prevent unwanted cracking but also to precisely guide the crack propagation. Both photomasks were 7″ soda-lime photomasks guaranteeing a minimum feature size of 5 with 0.5 μm tolerance and 2 μm position accuracy. The detailed photolithography conditions are provided in Supplementary Table . Replication of SU-8 pattern SU-8 micropatterns with cracking-assisted nanopatterns were replicated by using PUA (MINS-311RM, Minuta Tech., Osan, Korea) and polyethylene terephthalate film (Minuta Tech). The PUA solution was spin coated at 1,000 r.p.m. and cured using a handy-type ultraviolet lamp (365 nm, 4 W, UVL-21, Fisher Scientific Inc.) in a nitrogen environment for 2 min to minimize oxygen inhibition during photocuring. Both processed SU-8 pattern/mould and PUA are hydrophobic so that the micro/nanogap of the SU-8 pattern was easily filled with PUA by surface adhesion/affinity [26] . Then the additional PUA solution was poured and covered by a polyethylene terephthalate film, followed by photocuring to make the two PUA layers monolithic. After being peeled off from the SU-8 master, the PUA patterns were again used as moulds for PDMS (Sylgard 184 silicone elastomer kit, Dow Corning, USA) replica devices. Fabrication and handling of micro/nanofluidic device The roof-collapse problem of regular PDMS nanochannels on a glass substrate was resolved by using hard-PDMS (h-PDMS) with a relatively higher modulus (~9 N mm −2 ), which consists of VDT-731 (3.4 g, JSI Silicone, Seongnam, Korea), a Pt catalyst (18 μl, JSI silicone) and 2,4,6,8-tetramethyltetravinylcyclotetrasiloxane (4 μl, Sigma-Aldrich, Korea) [27] . The h-PDMS was spin coated at 1,000 r.p.m. on the PUA mould and cured in a hot oven (65 °C) for 30 min. Then, additional regular PDMS was poured onto the h-PDMS-coated mould, followed by curing in a hot oven (65 °C) for >4 h. It is noted that when a positive PUA mould was replicated with the h-PDMS, the h-PDMS precursor solution was well-degased in a vacuum jar approximately for an hour to avoid bubble generation. In addition, air bubbles trapped between the PUA (bottom) and the h-PDMS (top) surfaces during soft lithography floated up and disappeared while the h-PDMS and regular PDMS cured. Subsequently, the h-PDMS surfaces and a glass substrate were treated with oxygen plasma under 50 sccm of O 2 and 50 W for 30 s (Cute-MP, Femto Science, Korea) to make the surface hydrophilic and for strong irreversible bonding between them. Since the hybrid channel became hydrophilic, the micro/nanochannels could be automatically filled with aqueous solution (for example, water) by capillary forces as shown in Fig. 5f . The plasma treatment made the PDMS devices irreversibly bonded to the glass substrate, resulting in the tight sealing of the micro/nanochannels. The treatment also made all the channel surfaces hydrophilic so that aqueous solutions were flowed along the main microchannels easily and then towards the nanochanels. Air trapped in the nanochannels was easily eliminated by squeezing pressure driven by capillary forces and the high gas permeability of PDMS (5.2 × 10 −6 –3.4 × 10 −5 cm 2 s −1 ) (ref. 28 ). As a result, no air bubbles were formed in the device. Experimental set up and data analysis A ultraviolet intensity meter (SUSS MicroTec) was used to measure the exposure energy during the photolithography process. The thickness of the SU-8 film was measured using a surface profiler (P-6, KLA Tencor, USA). Atomic force microscopy (D3100, Veeco, USA) and scanning electron microscopy (Quanta200, FEI, USA) were used for imaging and quantifying cracks. An inverted fluorescence microscope (Ti-U, Nikon, Japan) equipped with a charge-couple device camera (ORCA R2, Hamamatsu Photonics, Japan) was used to obtain the optical and fluorescent microscopic images. FITC (Sigma-Aldrich) and fluorescently labelled microbeads (Invitrogen, USA) were used for visualizing and quantifying mass transport through nanochannels. Two pairs of 0.25-mm diameter platinum wires (Huntingdon, UK) were used as electrodes to apply electric potentials, which were generated and monitored via a source meter (Model No. 2635A, Keithley Instruments, USA). For data analysis and image processing, Image J (NIH, USA) and OriginPro 8 (OriginLab, USA) were used. How to cite this article: Kim, M. et al . Cracking-assisted photolithography for mixed-scale patterning and nanofluidic applications. Nat. Commun. 6:6247 doi: 10.1038/ncomms7247 (2015).